Directly converting CO2into a gasoline fuel The direct production of liquid fuels from CO 2 hydrogenation has attracted enormous interest for its significant roles in mitigating CO 2 emissions and reducing dependence on petrochemicals. Here we report a highly efficient, stable and multifunctional Na–Fe 3 O 4 /HZSM-5 catalyst, which can directly convert CO 2 to gasoline-range (C 5 –C 11 ) hydrocarbons with selectivity up to 78% of all hydrocarbons while only 4% methane at a CO 2 conversion of 22% under industrial relevant conditions. It is achieved by a multifunctional catalyst providing three types of active sites (Fe 3 O 4 , Fe 5 C 2 and acid sites), which cooperatively catalyse a tandem reaction. More significantly, the appropriate proximity of three types of active sites plays a crucial role in the successive and synergetic catalytic conversion of CO 2 to gasoline. The multifunctional catalyst, exhibiting a remarkable stability for 1,000 h on stream, definitely has the potential to be a promising industrial catalyst for CO 2 utilization to liquid fuels. For over 200 years, utilization of carbon-rich fossil fuels such as coal, oil and natural gas, has propelled the progress in human civilization, economic and social development [1] . However, the burning of fossil fuels gives rise to huge amounts of CO 2 emissions, which brings about adverse climate changes. Converting CO 2 from a detrimental greenhouse gas into value-added chemicals and fuels not only contributes to mitigating CO 2 emissions, but also provides valuable fuels and thus enhances energy security in light of the depletion of fossil resources and the strong fluctuation of oil prices [1] , [2] , [3] , [4] . Unfortunately, the activation of CO 2 and its hydrogenation to hydrocarbons or alcohols are challenging tasks because CO 2 is a fully oxidized, thermodynamically stable and chemically inert molecule [5] . Another challenge arises with the low C/H ratio obtained during CO 2 hydrogenation, due to the relatively low heat of CO 2 adsorption on catalyst surface [6] . This favors the fast hydrogenation of surface-adsorbed intermediates, leading to the formation of methane and a decrease in chain growth [6] . Most research to date, not surprisingly, is focusing on the selective hydrogenation of CO 2 to short-chain products, such as CO (refs 5 , 7 ), CH 3 OH (refs 8 , 9 , 10 ), HCOOH (ref. 11 ), CH 4 (ref. 12 ) and C 2 –C 4 olefins [13] , [14] , while few studies on long-chain hydrocarbons [15] , [16] . CO 2 can be hydrogenated to hydrocarbons by either direct or indirect route. The direct CO 2 hydrogenation (CO 2 -FT) is often described as the combination of the reduction of CO 2 to CO via reverse water-gas shift (RWGS) reaction and subsequent hydrogenation of CO to hydrocarbons via Fischer–Tropsch synthesis (FTS) [6] . The indirect route is often performed by using different reactors with syngas (a mixture of CO and H 2 , derived from coal, natural gas and biomass) and/or methanol intermediate formation [17] . In contrast, the direct route is more economic and environmentally benign while this approach usually yields CO and light paraffins as major products owing to weak CO hydrogenation activity and over-hydrogenation of olefins [18] . Gasoline-range hydrocarbons are generally produced from refining of petroleum, or from syngas via FTS process, or from methanol-to-gasoline (MTG) process [19] . So far, there has been no report on highly selective synthesis of gasoline from direct CO 2 hydrogenation. The key to this process is to search for a highly efficient catalyst. Owing to their excellent ability to catalyse both RWGS and FTS processes and high olefinic nature of obtained products, iron-based catalysts remain the preferred catalyst candidate for CO 2 -FT process [2] . Furthermore, density functional theory calculations have demonstrated that Fe 3 O 4 (111) surface is very capable of activating CO 2 (refs 20 , 21 ). Typically, iron catalysts need alkali metal promotion to attain desired activity and selectivity. It was reported that the addition of Na is beneficial to olefin production [22] , [23] , [24] . The existence of Na obviously enhances the surface basicity and carburization of iron-based catalyst, making the catalyst very active for CO 2 hydrogenation to light olefins [14] . Yet for the conventional iron-based catalysts, the hydrocarbon products generally follow the Anderson–Schulz–Flory (ASF) distribution, which is inherently wide and unselective [17] . More unfortunately, these hydrocarbons comprise mainly olefins and normal paraffins, with low octane number and unsuitable as gasoline fuel. Considering that zeolites are powerful in oligomerization/aromatization/isomerization of hydrocarbons due to their unique shape selectivity and acidity [17] , the combination of an iron-based CO 2 -FT catalyst with a zeolite into a multifunctional catalyst can shift product distribution towards high-octane gasoline-range isoparaffins and aromatics. In spite of considerable efforts made in the development of composite catalysts [15] , [18] , the selectivity to C 5+ hydrocarbons, especially centred C 5 –C 11 hydrocarbons, is not high enough owing to the poor coordination between the components of composite catalysts. In present work, we report a high efficient multifunctional catalyst comprised of Na–Fe 3 O 4 nanocatalyst and nanocrystalline HZSM-5 zeolite (Na–Fe 3 O 4 /HZSM-5 catalyst) for the direct conversion of CO 2 to gasoline-range hydrocarbons. This catalyst displays record selectivity towards C 5 –C 11 hydrocarbons (78%) as well as low CH 4 and CO selectivity under industrially relevant conditions. It was also discovered that the choice of active components and the integration manner of the components are crucial to control the product selectivity. CO 2 hydrogenation performance We initially prepared Na–Fe 3 O 4 nanocatalyst by a simple one-pot synthesis method and then applied it to CO 2 hydrogenation reaction. As shown in Fig. 1a , Na–Fe 3 O 4 catalyst exhibited 12% selectivity to CH 4 , 38% selectivity to C 5 –C 11 as well as a low CO selectivity (14%) at a CO 2 conversion of 34%. Notably, the hydrocarbon distribution followed a fairly linear trend for Na–Fe 3 O 4 , implying an ASF product distribution ( Fig. 1c ). In our quest for a compatible zeolite, a series of zeolites like HY, HBEA, HMOR, HZSM-23, HMCM-22 and HZSM-5, possessing the ability to catalyse olefin oligomerization reaction in varying degrees, were coupled with Na–Fe 3 O 4 catalyst for CO 2 hydrogenation. 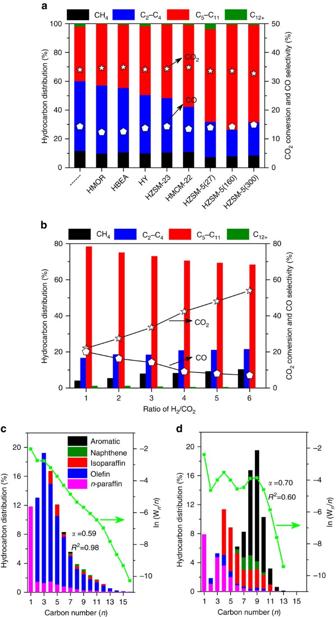Figure 1: Catalytic performance for CO2hydrogenation. (a) CO2conversion and product selectivity over different Na–Fe3O4/Zeolite catalysts; reaction conditions: H2/CO2=3,320 °C, 3 MPa and 4,000 ml h−1gcat−1. (b) CO2conversion and product selectivity at different H2/CO2ratios over Na–Fe3O4/HZSM-5(160) catalyst at 320 °C, 3 MPa and 4,000 ml h−1gcat−1. (c,d) The detailed hydrocarbon product distribution obtained over Na–Fe3O4(c) and Na–Fe3O4/HZSM-5(160) (d) catalysts, an additional ASF plot andαvalue comparison of above two catalysts are also depicted;Wnis the weight fraction of a product withncarbon atoms. The description of zeolite channels and NH 3 -TPD results were listed in Supplementary Table 1 and Supplementary Fig. 1 . As shown in Fig. 1a , CO 2 conversion and CO selectivity are not obviously related to zeolite type, predominantly decided by the first component of Na–Fe 3 O 4 , whereas the distribution of hydrocarbon products is evidently influenced by the zeolite pore structure on Na–Fe 3 O 4 /Zeolite catalysts for CO 2 hydrogenation. It is noteworthy that three types of zeolites with 10 member ring (MR) channels exhibit higher C 5 –C 11 selectivities in the order of HZSM-5 (3-dimensional)>HMCM-22 (2-dimensional)>HZSM-23 (1-dimensional). This result suggests zeolites with 10 MR channels can favour the oligomerization of olefins and the production of C 5 –C 11 hydrocarbons. Besides the pore structure, the acidity, which is depended on the SiO 2 /Al 2 O 3 ratio of zeolite, is another important factor affecting hydrocarbon distribution. It suggests that the stronger acidity of HZSM-5(27) could cause the over-cracking of heavy hydrocarbons to C 1 –C 4 hydrocarbons, whereas the weaker one of the HZSM-5(300) is not beneficial to the oligomerization/isomerization/aromatization of primary CO 2 -FT products, thus both disfavour the selective production of C 5 –C 11 hydrocarbons ( Fig. 1a ). In summary, HZSM-5(160) zeolite is suitable for C 5 –C 11 hydrocarbon synthesis due to the presence of medium/strong acid sites and 3-dimensional pore structure. Figure 1: Catalytic performance for CO 2 hydrogenation. ( a ) CO 2 conversion and product selectivity over different Na–Fe 3 O 4 /Zeolite catalysts; reaction conditions: H 2 /CO 2 =3,320 °C, 3 MPa and 4,000 ml h −1 g cat −1 . ( b ) CO 2 conversion and product selectivity at different H 2 /CO 2 ratios over Na–Fe 3 O 4 /HZSM-5(160) catalyst at 320 °C, 3 MPa and 4,000 ml h −1 g cat −1 . ( c , d ) The detailed hydrocarbon product distribution obtained over Na–Fe 3 O 4 ( c ) and Na–Fe 3 O 4 /HZSM-5(160) ( d ) catalysts, an additional ASF plot and α value comparison of above two catalysts are also depicted; W n is the weight fraction of a product with n carbon atoms. Full size image The Na–Fe 3 O 4 /HZSM-5(160) multifunctional catalyst provided a CO 2 conversion of 34% and selectivities to CH 4 , C 2 –C 4 , C 5 –C 11 and C 12+ hydrocarbons of 8, 18, 73 and 1%, respectively, under 320 °C, 3 MPa, and H 2 /CO 2 ratio of 3 ( Fig. 1a ). Moreover, when the H 2 /CO 2 ratio of feed gas was switched to 1, we observed an even higher selectivity to gasoline fraction (78%) and only 4% CH 4 with a CO 2 conversion of 22% over Na–Fe 3 O 4 /HZSM-5(160) catalyst ( Fig. 1b ). 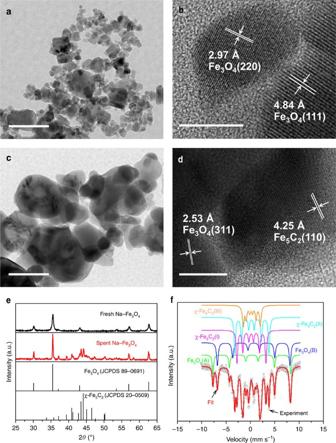Figure 2: Structural characterization of Na–Fe3O4catalyst. (a,c) TEM images of fresh (a) and spent (c) Na–Fe3O4catalyst. Scale bar, 100 nm. (b,d) HRTEM images of fresh (b) and spent (d) Na–Fe3O4catalyst. Scale bar, 10 nm. (e) XRD patterns of fresh and spent Na–Fe3O4catalyst. (f) Mössbauer spectra of spent Na–Fe3O4catalyst. To our knowledge, this is the highest selectivity for gasoline-range hydrocarbons reported for CO 2 hydrogenation ( Supplementary Table 2 ). A higher H 2 /CO 2 ratio benefits CO 2 conversion, which rose to 54% at H 2 /CO 2 =6, for instance, whereas it disfavours the selective formation of gasoline fraction. Selectivities varied in the range from 68 to 78% for C 5 –C 11 and 4 to 10% for CH 4 in the investigated H 2 /CO 2 ratio (1 to 6). To further elucidate the function of HZSM-5, a detailed product distribution has been done on Na–Fe 3 O 4 /HZSM-5(160) catalyst ( Fig. 1d ). Compared with Na–Fe 3 O 4 catalyst ( Fig. 1c ), the use of HZSM-5 as the second component significantly decreased the selectivities to CH 4 and C 2 –C 4 , and altered the product distribution towards gasoline-range isoparaffins and aromatics. 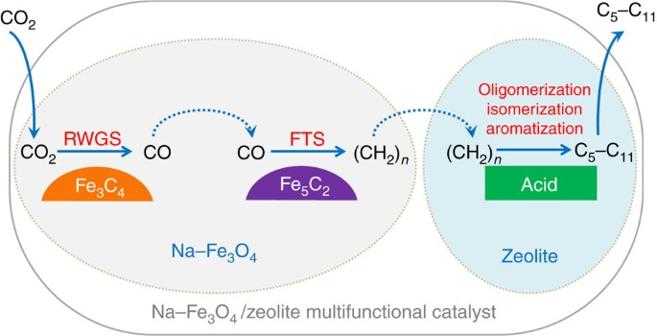Figure 3: Reaction scheme for CO2hydrogenation to gasoline-range hydrocarbons. The CO2hydrogenation reaction over Na–Fe3O4/Zeolite multifunctional catalyst takes place in three steps: (1) an initially reduced to CO intermediate via RWGS, (2) a subsequent hydrogenation of CO to α-olefins intermediate via FTS and (3) the formation of gasoline-range hydrocarbons via the acid-catalysed oligomerization, isomerization and aromatization reactions. Moreover, oxygenates formation is inhibited at the presence of zeolite ( Supplementary Table 3 ). An additional ASF plot and the probability of chain growth ( α ) value comparison of above two catalysts are also given in Fig. 1c,d . Relatively, Na–Fe 3 O 4 /HZSM-5 catalyst exhibited an α value of 0.70, higher than that of 0.59 for Na–Fe 3 O 4 catalyst, confirming that the production of long-chain hydrocarbons was promoted on the multifunctional catalyst. The product distribution on the multifunctional catalyst deviated greatly from the typical ASF distribution, which could be attributed to the secondary reactions, such as oligomerization, isomerization and aromatization, occurring on zeolite acid sites. Further, a tunable isoparaffin/aromatic ratio in gasoline-range hydrocarbons is achieved by simply altering zeolite type ( Supplementary Fig. 2 ). Under the same conditions, HZSM-5(27), HZSM-5(160) and HZSM-5(300) with MFI topology produced higher amount of aromatics (up to 61% of aromatics in gasoline fraction) while HMCM-22 with MWW topology produced mainly isoparaffins (46% of isoparaffins in gasoline fraction). This phenomenon has a close correlation with the topology of different zeolites. HMCM-22 zeolite with 10 MR pore openings has a unique lamellar structure consisting of two independent pore systems, which leads to HMCM-22 with potential catalytic properties in isomerization, alkylation and disproportionation [25] . 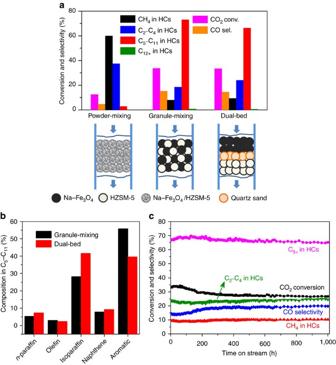Figure 4: CO2hydrogenation performance over the multifunctional catalysts with different proximity. (a) CO2conversion and product selectivity over different combinations of Na–Fe3O4and HZSM-5 catalysts conducted at the same reaction conditions asFig. 1a; HCs: hydrocarbons. (b) The composition of gasoline-range hydrocarbons on different Na–Fe3O4/HZSM-5(160) composite catalysts. (c) The stability of the Na–Fe3O4/HZSM-5 catalyst with dual-bed configuration under the same reaction conditions asFig. 1a. The hydrocarbon selectivities are normalized with the exception of CO. In addition, the major aromatics produced over Na–Fe 3 O 4 /HZSM-5 catalyst, were identified to be toluene, xylene, ethyltoluene, trimethylbenzene and dimethyl ethylbenzene, while less benzene and durene formed (both <1% in gasoline) ( Supplementary Table 4 ). Such aromatic product distribution is evidently different from that derived from MTG process. It will not need an extra separation process usually applied in MTG process due to the higher content of durene in gasoline. Structural characterization To reveal the nature of active sites that favors the formation of gasoline-range hydrocarbons, we resorted to multiple characterization techniques to investigate the structure of multifunctional catalyst. Na–Fe 3 O 4 catalyst was composed of nanosized Fe 3 O 4 with an average size of 13.1 nm, and the residual Na (0.7 wt%, determined by inductively coupled plasma (ICP)) was well distributed on the surface of Fe 3 O 4 nanoparticles, with no obvious segregation ( Fig. 2a,b,e ; Supplementary Figs 3 and 4e ). HZSM-5(160) was highly crystalline and appeared to be cuboid crystals ranged from 200 to 500 nm ( Supplementary Fig. 4 ). Characterization of high resolution transmission electron microscopy (HRTEM), X-ray diffraction (XRD) and Mössbauer spectra showed that two different types of iron phase were discerned in the spent Na–Fe 3 O 4 catalyst, with 32.4% of Fe 3 O 4 and 67.6% of χ-Fe 5 C 2 phase ( Fig. 2c–f ; Supplementary Table 5 ). Metallic iron is formed when Na–Fe 3 O 4 is reduced in H 2 prior to reaction ( Supplementary Fig. 4c ). Upon exposure of the catalyst to the reaction atmosphere, Fe 5 C 2 and Fe 3 O 4 are formed as a result of the interaction of metallic iron with carbon and oxygen species from the dissociated carbon oxides [26] . Appropriate proportion and arrangement of Fe 3 O 4 (active sites for RWGS) and Fe 5 C 2 (active sites for FTS) [26] , we speculated, is responsible for low CO selectivity (lower than 20%) with relatively high CO 2 conversion during CO 2 hydrogenation. Figure 2: Structural characterization of Na–Fe 3 O 4 catalyst. ( a , c ) TEM images of fresh ( a ) and spent ( c ) Na–Fe 3 O 4 catalyst. Scale bar, 100 nm. ( b , d ) HRTEM images of fresh ( b ) and spent ( d ) Na–Fe 3 O 4 catalyst. Scale bar, 10 nm. ( e ) XRD patterns of fresh and spent Na–Fe 3 O 4 catalyst. ( f ) Mössbauer spectra of spent Na–Fe 3 O 4 catalyst. Full size image Reaction scheme for CO 2 hydrogenation In the basis of the results above, we propose a reaction scheme of CO 2 hydrogenation to hydrocarbons over Na–Fe 3 O 4 /Zeolite multifunctional catalyst as illustrated in Fig. 3 . This scheme indicates that the multifunctional catalyst, with three types of active sites, exhibits complementary and compatible properties. During CO 2 hydrogenation, CO 2 is initially reduced to CO by H 2 via RWGS on Fe 3 O 4 sites, followed by a subsequent hydrogenation of CO to α-olefins via FTS on Fe 5 C 2 sites. The olefin intermediates generated on the iron-based catalyst then diffuse to zeolite acid sites, on which they undergo acid-catalysed reactions (oligomerization, isomerization and aromatization), as a consequence, the gasoline-range isoparaffins and aromatics are selectively formed and finally diffuse out of zeolite pores. Besides, CO 2 conversion and product selectivity could be modulated by varying the mass ratio of Na–Fe 3 O 4 relative to zeolite ( Supplementary Fig. 5 ), which provides further support to the above hypothesis that Na–Fe 3 O 4 /Zeolite catalyst is multifunctional and the reaction involves intermediate migration among different active sites. Figure 3: Reaction scheme for CO 2 hydrogenation to gasoline-range hydrocarbons. The CO 2 hydrogenation reaction over Na–Fe 3 O 4 /Zeolite multifunctional catalyst takes place in three steps: (1) an initially reduced to CO intermediate via RWGS, (2) a subsequent hydrogenation of CO to α-olefins intermediate via FTS and (3) the formation of gasoline-range hydrocarbons via the acid-catalysed oligomerization, isomerization and aromatization reactions. Full size image Proximity effect in multifunctional catalysts The proximity of the two components in multifunctional catalysts has been reported to exert significant influence on catalytic activity (refs 27 , 28 , 29 ). In our case, we found that it is also vital for selective conversion of CO 2 to hydrocarbons ( Fig. 4a ). When Na–Fe 3 O 4 and HZSM-5 were integrated by powder mixing, the closest proximity between iron-based sites and zeolite acid sites turned out to be detrimental, exhibiting a very low CO 2 conversion (13%) and high undesired CH 4 selectivity up to 60%. The reason, we speculated, is that the zeolite acid sites poison the Na-induced alkali sites on the Fe 3 O 4 surface, leading to a decrease in the surface basicity and carburization degree of Fe 3 O 4 catalyst. Likewise, another 2%Na–10%Fe/HZSM-5 catalyst with a close intimacy we prepared by an incipient wetness impregnation method as a comparison also presented a poor performance on CO 2 hydrogenation ( Supplementary Table 3 ). When Na–Fe 3 O 4 and HZSM-5 were combined by granule mixing, the distance between iron-based and zeolite acid sites was enlarged, and the olefin intermediates formed on iron-based sites diffused through wide pores to zeolite, where they immediately underwent oligomerization, isomerization and aromatization reactions, giving rise to the highest C 5 –C 11 selectivity (73%) at a CO 2 conversion of 34%. It demonstrated an appropriate distance between iron-based and acid sites is critical for achieving excellent performance. With regard to dual-bed configuration, where HZSM-5 was packed below Na–Fe 3 O 4 and separated by a thin layer of inert quartz sand, the distance between iron-based and acid sites got larger. It exhibited a slightly lower C 5 –C 11 selectivity (67%) and the same CO 2 conversion as the manner of granule mixing. Figure 4: CO 2 hydrogenation performance over the multifunctional catalysts with different proximity. ( a ) CO 2 conversion and product selectivity over different combinations of Na–Fe 3 O 4 and HZSM-5 catalysts conducted at the same reaction conditions as Fig. 1a ; HCs: hydrocarbons. ( b ) The composition of gasoline-range hydrocarbons on different Na–Fe 3 O 4 /HZSM-5(160) composite catalysts. ( c ) The stability of the Na–Fe 3 O 4 /HZSM-5 catalyst with dual-bed configuration under the same reaction conditions as Fig. 1a . The hydrocarbon selectivities are normalized with the exception of CO. Full size image Note that the composition of gasoline-range hydrocarbons also relies on different combinations of Na–Fe 3 O 4 and HZSM-5 catalysts ( Fig. 4b ). It is inclined to produce more aromatics under the manner of granule mixing, while more isoparaffins are produced under the dual-bed configuration. We have further measured the stability of the Na–Fe 3 O 4 /HZSM-5 catalyst with dual-bed configuration ( Fig. 4c ). It demonstrated good stability over 1,000 h on stream. The C 5+ selectivity stably maintained at 67±2% throughout the test. CO 2 conversion was only reduced by 6% within the first 300 h on stream, related to the loss of active Fe surface as a result of the sintering of iron taken place during this stage ( Fig. 2c ) [30] . Afterwards, the iron species tended to be stable and thus CO 2 conversion was constant during the next few hundred hours. The total coke deposit on HZSM-5 was only 3.7 wt% ( Supplementary Fig. 6 ). Thus, the present multifunctional catalyst is stable and suitable for the direct conversion of CO 2 to gasoline. In conclusion, we have succeeded in preparing a highly selective Na–Fe 3 O 4 /HZSM-5 multifunctional catalyst for the direct production of gasoline from CO 2 hydrogenation. This catalyst enables RWGS over Fe 3 O 4 sites, olefin synthesis over Fe 5 C 2 sites, and oligomerization/aromatization/isomerization over zeolite acid sites. The concerted action of the active sites calls for precise control of their structures and proximity. It exhibited 78% selectivity to C 5 –C 11 as well as low CH 4 and CO selectivity, and gasoline fraction are mainly isoparaffins and aromatics thus favoring the octane number. Moreover, the composition of C 5 –C 11 can be tuned by the choice of zeolite type and the integration manner of multifunctional catalyst. In particular, this multifunctional catalyst and the process may allow use of the feed gas with a low H 2 /CO 2 ratio thus reduce the cost of hydrogen. This study paves a new path for the synthesis of liquid fuels by utilizing CO 2 and H 2 . Furthermore, it provides an important approach for dealing with the intermittency of renewable sources (sun, wind and so on) by storing energy in liquid fuels. Catalyst preparation We prepared the Na–Fe 3 O 4 nanocatalyst by a one-pot synthesis method. Typically, 31.62 g FeCl 3 ·6H 2 O and 12.54 g of FeCl 2 ·4H 2 O were added to 150 ml deionized (DI) water containing 5.1 ml of 12.1 mol l −1 HCl with stirring to form a clear solution. In the above solution, 1.5 mol l −1 of NaOH was then added dropwise under stirring at 60 °C. Consequently, an instant black precipitate was generated, and the pH value of final suspension was maintained at 10. The resulting suspension was kept with stirring for 1 h. The product was separated by a magnet, and washed once with 800 ml of DI water to obtain a Fe 3 O 4 nanocatalyst modified with a certain content of residual Na. The fresh-made nanocatalyst was dried overnight at 60 °C and directly used for CO 2 hydrogenation reaction without further thermal treatment to maintain their nanostructure and morphology. The chemical reaction for synthesis of Fe 3 O 4 is given by equation (1) [31] . In the above synthesis, we prepared and modified the catalysts simultaneously without any extra steps. NaOH is served as not only the precipitating agent but also the promoter source. By changing the number of washing times and the volume of water consumption for each wash, the content of promoter can be regulated easily. For comparison, a Fe 3 O 4 nanocatalyst without Na modification was prepared by the same method just substituting NH 3 ·H 2 O (5 wt%) for NaOH (1.5 mol l −1 ) as the precipitating agent. HY (SiO 2 /Al 2 O 3 =5), HMCM-22 (SiO 2 /Al 2 O 3 =30) and HZSM-5 zeolites (SiO 2 /Al 2 O 3 =27, 160, 300) were commercially available from Nankai University catalyst company, China. HBEA (SiO 2 /Al 2 O 3 =25) and HMOR (SiO 2 /Al 2 O 3 =20) were purchased from Zeolyst International. HZSM-23 (SiO 2 /Al 2 O 3 =80) was synthesized by a hydrothermal method [32] . Before used, the zeolites were calcined in air at 500 °C for 4 h. The Na–Fe 3 O 4 /Zeolite catalyst was typically prepared by granule mixing Na–Fe 3 O 4 catalyst with zeolite at a mass ratio of the two components of 1:1 unless otherwise noted. Take the preparation of Na–Fe 3 O 4 /HZSM-5 catalyst with granule mixing as an example. Na–Fe 3 O 4 and HZSM-5 were pressed into pellets (30 MPa), crushed and sieved to 20–40 meshes (granule sizes of 380–830 μm), respectively. Then, the granules of the two samples were mixed together by shaking in a vessel. For preparation of Na–Fe 3 O 4 /HZSM-5 catalyst with powder mixing ( Fig. 4a ), Na–Fe 3 O 4 and HZSM-5 were mixed in an agate mortar for 2 min, and then pressed, crushed and sieved to 20–40 meshes. The obtained sample was denoted as Na–Fe 3 O 4 /HZSM-5-PM. For comparison, 2 wt% Na–10 wt% Fe/HZSM-5(160) catalyst was prepared by incipient wetness impregnation with aqueous Fe(NO 3 ) 3 and NaNO 3 in addition. After impregnation for 12 h, the samples were dried at 60 °C for 8 h and calcined at 500 °C for 4 h. Catalyst characterization The Na content of the Na–Fe 3 O 4 nanocatalyst was analysed with an inductively coupled plasma optical emission spectrometer (ICP-OES, Perkin-Elmer Optima 7300DV) after the catalyst sample had been digested with hydrochloric acid at room temperature. XRD spectra of the powder catalysts were recorded with a PANalytical X’Pert Pro diffractometer using Cu-Kα (40 kV, 40 mA) irradiation. For the XRD test of the reduced catalysts, passivation treatment with 1% O 2 /99% N 2 at room temperature was conducted after reduced at 350 °C for 8 h in H 2 . The specific surface area of the catalysts was analysed by the BET method carrying out N 2 adsorption measurements at −196 °C on a Quantachrome instrument. All the samples were degassed at 300 °C for 6 h under vacuum before adsorption. The morphology of the catalysts was characterized by scanning electron microscopy (SEM) on a JSM-7800F microscope operated at an accelerating voltage of 1.5 kV. Transmission electron microscopy (TEM) images were obtained on a JEM-2100 system (JEOL) with an acceleration voltage of 200 kV. The samples were ultrasonically suspended in ethanol and placed onto a carbon film supported over a Cu grid for that purpose. NH 3 temperature-programmed desorption (NH 3 -TPD) measurements were performed on a home-made setup. Typically, 100 mg sample was loaded into a U-shaped quartz microreactor (i.d.=4 mm) and pretreated at 600 °C for 0.5 h in flowing He. After pretreatment, the sample was cooled down to 100 °C and saturated with NH 3 . The sample was flushed in He flow for 0.5 h to remove the gas phase NH 3 . Then, NH 3 -TPD was carried out in a constant flow of He (30 ml min −1 ) from 100 to 700 °C at a heating rate of 10 °C min −1 . The concentration of NH 3 in the exit gas was continuously detected by a gas chromatograph (SHIMADZU) with a thermal conductivity detector (TCD). Thermo-gravimetric and differential thermal analyses (TG–DTA) of zeolite samples were performed on a Perkin-Elmer Diamond TGS-2 and DTA1700 apparatus. The experiments were carried out in the temperature range of 30–1,000 °C, with a heating rate of 10 °C min −1 in flowing air (40 ml min −1 ). The 57 Fe Mössbauer spectra (MES) of the catalysts were carried out on a Topologic 500A spectrometer driving with a proportional counter at room temperature. The radioactive source was 57 Co (Rh) moving in a constant acceleration mode. Data analyses were performed assuming a Lorentzian lineshape for computer folding and fitting. The components of iron phases were identified based on their Mössbauer parameters including isomer shift, quadruple splitting and magnetic hyperfine field. Catalytic performance tests CO 2 hydrogenation reactions were performed in a stainless steel fixed-bed reactor with an inner diameter of 14 mm. Typically 1 g of composite catalyst (20–40 meshes) with Na–Fe 3 O 4 /Zeolite=1/1 (mass ratio) was used unless otherwise stated. Prior to reaction, the catalyst was in-situ reduced at 350 °C for 8 h in a pure H 2 flow at atmospheric pressure. After reduction, the reactor was cooled to 320 °C. Then the reactant gas mixture H 2 /CO 2 /N 2 (containing 4 vol% N 2 as the internal standard) was fed into the reactor, and the system was pressured gradually to 3 MPa. All of the products from the reactor were introduced in a gaseous state and analysed with two online gas chromatographs (GC) (VARIAN 3800). N 2 , CO, CO 2 and CH 4 were analysed using a GC system equipped with a TCD, a Hayesep C column and a molecular sieve 13X column. The organic compounds including hydrocarbons and oxygenates were analysed using another GC system equipped with a flame ionization detector (FID) and a PONA capillary column. The reaction was carried out under the conditions of H 2 /CO 2 =3,320 °C, 3 MPa and 4,000 ml h −1 g cat −1 unless otherwise stated. For a test with Na–Fe 3 O 4 only of Fig. 1a , 0.5 g of catalyst was used, and the flow rate of feed gas is 4,000 ml h −1 . Moreover, the hydrocarbon distribution was calculated based on the total carbon moles with a unit of C-mol% on all tested catalysts. The carbon balances of various reactions were calculated, which were over 95% for all reactions. The catalytic performances after at least 2 h on stream were typically used for discussion. CO 2 conversion was calculated by equation (2): where CO 2 in and CO 2 out represent the molar fraction of CO 2 at the inlet and outlet, respectively. CO selectivity was calculated according to equation (3): where CO out represents the molar fraction of CO at the outlet. The selectivity of different hydrocarbon in total hydrocarbons was given as equation (4): Data availability The data supporting the findings of this study are available within the article and its Supplementary Information files. All other relevant source data are available from the corresponding author upon reasonable request. How to cite this article: Wei, J et al . Directly converting CO 2 into a gasoline fuel. Nat. Commun. 8 , 15174 doi: 10.1038/ncomms15174 (2017). Publisher’s note: Springer Nature remains neutral with regard to jurisdictional claims in published maps and institutional affiliations.